Double-heterojunction nanorods As semiconductor heterostructures play critical roles in today’s electronics and optoelectronics, the introduction of active heterojunctions can impart new and improved capabilities that will enable the use of solution-processable colloidal quantum dots in future devices. Such heterojunctions incorporated into colloidal nanorods may be especially promising, since the inherent shape anisotropy can provide additional benefits of directionality and accessibility in band structure engineering and assembly. Here we develop double-heterojunction nanorods where two distinct semiconductor materials with type II staggered band offset are both in contact with one smaller band gap material. The double heterojunction can provide independent control over the electron and hole injection/extraction processes while maintaining high photoluminescence yields. Light-emitting diodes utilizing double-heterojunction nanorods as the electroluminescent layer are demonstrated with low threshold voltage, narrow bandwidth and high efficiencies. Semiconductor nanocrystals or colloidal quantum dots (CQDs) and their heterostructures that can be synthesized by versatile solution chemistry are being considered for advancing multiple areas of technology [1] , [2] . In particular, core/shell heterostructures with type I straddling band offset exhibiting high photoluminescence (PL) quantum yields show much promise in imaging [3] , lighting [4] , [5] and display [6] , [7] , [8] , [9] , [10] , [11] applications. Although type II staggered band offset materials have also been achieved and have been shown to allow efficient photoinduced charge separation [12] , [13] , [14] , [15] , [16] and improved light amplification [17] , [18] , to date, the highly luminescent type I core/shell heterostructure is the predominant choice in emerging nanocrystal-based products. However, the type I core/shell structure may be less than ideal especially in photovoltaics, optoelectronics and related device applications in that the large band gap shell prohibits physical access to the core and poses a significant barrier for carrier injection and extraction [19] . In general, the ability to effectively control the direction, separation and recombination of charge carriers while minimizing power consumption is central to high-performance energy-efficient electronic/optoelectronic devices. In the current state-of-the-art optoelectronics, controlling band alignment/offset via epitaxially well-defined heterostructures is a ubiquitous solution for such purposes. Of special note is the double heterostructure where a smaller band gap semiconductor is sandwiched between wider band gap materials [20] , [21] . Double heterojunctions can provide efficient carrier injection, low threshold voltage and reduced heating, allowing increased output/performance before reaching thermal limitations [22] . The double heterostructure has enabled semiconductor lasers and is now widely used in LEDs and bipolar transistors among many devices [20] , [21] , [23] , [24] . Introducing structurally and electronically well-defined double or multiple heterojunctions within a nanocrystal may lead to analogous benefits and facilitate utilization of unique characteristics of CQDs. Here, we develop double-heterojunction nanorods (DHNRs) where two larger band gap semiconductor materials with type II band offset surround and are both in physical contact with a smaller band gap QD-emitting center. This structure can facilitate independent control over the electron and hole injection/extraction processes while maintaining high PL quantum yields and solution processability. We demonstrate the utility of introducing active heterojunctions in CQDs by fabricating LEDs that utilize our DHNRs as the electroluminescent layer. These DHNR LEDs exhibit brightness over 30,000 cd m −2 and maximum external quantum, current and power efficiencies of 2.6%, 5.70 cd A −1 and 6.26 lm W −1 , respectively, surpassing the performance of type I core/shell QD LEDs of similar device architecture. Challenges in synthesis Achieving DHNRs that are analogous to epitaxial thin-film double heterostructures requires the growth of two distinct larger band gap materials that would form type II band offset by themselves (or p- and n-doped materials) surrounding one semiconductor. In the thin-film geometry, deposition onto a substrate allows symmetry breaking and the sequential growth inherently leads to the middle component being interfaced with two different materials. In the solution synthesis of CQDs, such a growth becomes challenging because the ‘substrate’ is a soluble particle that may often prefer a surface area-reducing core/shell type structure, and therefore, means of growth that is spatially selective must be imposed for each added component. Recent advances in the synthesis of multi-component semiconductor nanocrystals with anisotropic shapes/morphologies [25] , [26] , [27] , [28] , [29] , [30] provide a potential solution. When combined with band alignment/band gap engineering of semiconductor heterostructures, anisotropic nanorods can also provide control over both spatial and electronic directionality and accessibility [12] , [13] , [14] , [15] , [31] , [32] (for example, for efficient charge injection/extraction). However, to achieve our envisioned DHNRs, there are additional difficulties. For example, the two larger band gap materials are likely to be better lattice matched with each other than with the smaller gap material leading to unwanted interfaces. Imposing growth to be only along the rod axis can lead to double heterojunctions in collinear structures, but the smaller gap emitting materials will have partially exposed surfaces limiting desired characteristics such as high PL yields. These challenges associated with DHNR growth, thus far, have not been addressed using solution chemistry, but the ability to epitaxially grow two distinct materials around a nanocrystal should in general lead to a whole new subclass of complex nanomaterials with multiple functionalities. Photocatalytic activity and luminescence upconversion enabled by metal [33] and a semiconductor of different composition [34] grown at the tip of a dot-in-a-rod structure, respectively, demonstrate promise in such directions of materials synthesis. Multiple compositions in nanorod heterostructures or hybrid structures may lead to additional opportunities such as unique means of assembly [35] . Our approach to DHNRs combines the preferential growth along [001] direction of wurtzite semiconductor nanorods with core/shell-like growth. 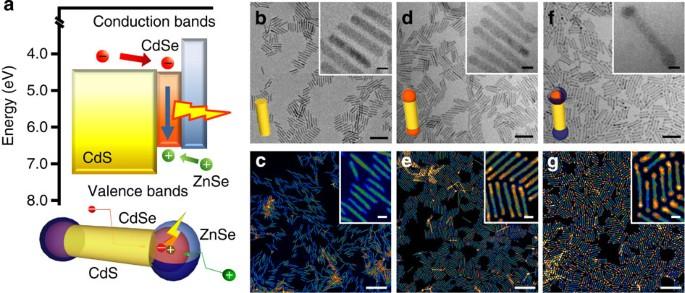Figure 1: Double-heterojunction nanorods (DHNRs). (a) Energy band diagram and schematic of the geometric structure of DHNRs consisting of type II band offset CdS and ZnSe both in contact with the emitting smaller band gap CdSe quantum dot. (b–g) Representative TEM and STEM images of CdS nanorod seeds (b,c), CdS/CdSe nanorod heterostructures (d,e) and CdS/CdSe/ZnSe DHNRs (f,g). Electron microscopy images show the shape evolution during each step of the formation of DHNRs. Scale bar, 50 nm forb,dandf(insets: 5 nm) and 100 nm forc,eandg(insets: 10 nm). The average tip diameter changes from 4.2 to 5.5 nm on ZnSe growth corresponding to ~2 to 3 monolayers of ZnSe. Figure 1a shows the band diagram and the schematic of DHNRs synthesized here, where CdSe is interfaced with both CdS and ZnSe. CdSe, which forms type I band offset with both CdS and ZnSe, becomes the emitting/charge recombination center. CdS and ZnSe form type II band offset and can facilitate electron and hole injection, respectively. Their band alignment should also make these two outer layer materials useful for blocking opposite charge carriers. The synthesis of DHNRs begins with CdS nanorods ( Fig. 1b,c ) followed by selective growth of CdSe at the tips ( Fig. 1d,e ) much like the barbell or rod/rod/rod shaped type II nanorod heterostructures of CdTe/CdSe/CdTe that have been reported previously [13] , [14] , [36] . The key distinction and thus the main challenge here is the selective growth of the third component, ZnSe. By optimizing reaction temperature and time as well as the amount of ZnSe precursors, the desired selective growth of ZnSe on CdSe ( Fig. 1f,g ) can be achieved while maintaining the tight size distribution of the initial CdS nanorods. Considering the lattice mismatch, which is the largest between CdSe and ZnSe (~7%), this selective growth may be surprising and therefore should be analysed in further detail as we discuss below. Nevertheless, since the net change in the surface/interface energy rather than lattice strain alone dictates the overall energy of the system, we suspect that lower surface energy of the exposed CdS facets leads to this preferential growth on CdSe tips [37] , [38] , [39] . Figure 1: Double-heterojunction nanorods (DHNRs). ( a ) Energy band diagram and schematic of the geometric structure of DHNRs consisting of type II band offset CdS and ZnSe both in contact with the emitting smaller band gap CdSe quantum dot. ( b – g ) Representative TEM and STEM images of CdS nanorod seeds ( b , c ), CdS/CdSe nanorod heterostructures ( d , e ) and CdS/CdSe/ZnSe DHNRs ( f , g ). Electron microscopy images show the shape evolution during each step of the formation of DHNRs. Scale bar, 50 nm for b , d and f (insets: 5 nm) and 100 nm for c , e and g (insets: 10 nm). The average tip diameter changes from 4.2 to 5.5 nm on ZnSe growth corresponding to ~2 to 3 monolayers of ZnSe. Full size image Structural characterization Characterization of selective growth of ZnSe on CdSe is arguably as important as the optimum synthesis conditions, and multiple independent techniques should be utilized to confirm the composition and structure. Transmission electron microscopy (TEM) and scanning TEM (STEM) images as exemplified in Fig. 1f,g shows that the rod/rod/rod shape of CdSe/CdS/CdSe changes to a more barbell-like structure on ZnSe growth. This ripening of the tips is consistent with the expected selective growth on CdSe. The average diameter changes from 4.2 to 5.5 nm at the tips, whereas it remains nearly constant at the center of the rods (change of ~0.5 nm or less). There is also an increase in the average overall length of ~3 nm, suggesting a growth of shell-like ZnSe over CdSe. Energy dispersive X-ray spectroscopy (EDS) results also show considerable amount of Zn (~12%) with an increased Se content verifying growth of ZnSe (see Supplementary Fig. 1 ). EDS analysis using aberration-corrected STEM to map composition at different regions of DHNRs shows that Zn and Se are concentrated at the tips and S at the center, whereas Cd is uniformly spread throughout the DHNRs (see Supplementary Fig. 2 ). Powder X-ray diffraction (XRD) also shows evidence of selective ZnSe growth. The XRD patterns of DHNRs at each step of the synthesis are shown in Fig. 2 . Distinctive and sharp (002) peak of CdS does not change despite CdSe growth, indicating that CdSe grows along the c axis of CdS nanorods. As CdSe grows, additional peaks at smaller 2 θ values than the corresponding CdS peaks appear as expected of a larger lattice material of same crystal structure. The final step of ZnSe growth is difficult to detect with XRD, given the average of ~2- to 3-monolayer thickness expected from TEM and STEM images. The changes in XRD peak positions (from curve fitting in Fig. 2 ) show an interesting result that supports selective growth of ZnSe. Peaks corresponding to CdS do not change appreciably, but CdSe peaks are up-shifted significantly. The up-shifts correspond to a lattice constant decrease of ~0.1% (or an insignificant change) for CdS, whereas CdSe exhibits an order of magnitude larger than ~1.1% decrease after ZnSe growth (see Supplementary Table 1 ). What this result implies is that ZnSe growth places only CdSe under compressive strain owing to the lattice mismatch. This decrease only in the CdSe lattice constant provides another important evidence for selective ZnSe growth. 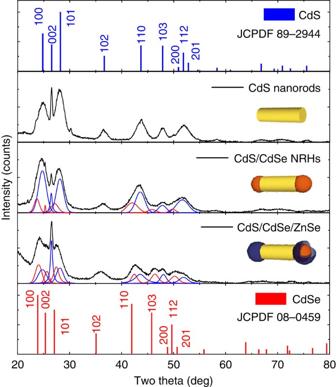Figure 2: X-ray diffraction patterns from each step of DHNR synthesis. The selective shifts in the CdSe peaks as analyzed by curve fitting shown indicate selective growth of ZnSe on CdSe necessary to achieve the desired double heterojunctions. Figure 2: X-ray diffraction patterns from each step of DHNR synthesis. The selective shifts in the CdSe peaks as analyzed by curve fitting shown indicate selective growth of ZnSe on CdSe necessary to achieve the desired double heterojunctions. Full size image To characterize composition distribution in the DHNRs with near atomic resolution, high-angle annular dark field (HAADF) imaging was carried out on an aberration-corrected STEM. Heavier elements have larger electron scattering cross-sections at high angles and thus higher intensity in the Z-contrast images. The atomic column resolution of Z-contrast afforded by the aberration-corrected STEM can therefore reveal composition variations within individual DHNRs, allowing identification of heterointerfaces with near atomic precision. High-resolution HAADF STEM image in Fig. 3a shows a tip of a DHNR consisting of CdS/CdSe barbell structure with a thin ZnSe layer (ZnSe thickness was controlled by the amount of Se added, 0.1 mmol in this case). The scattering intensity for each cation–anion column pair is always larger for the cation in the central part of the tip ( Fig. 3b , curve b1). This intensity difference is expected of CdSe since the cation is the heavier element. In contrast, there are several cases that exhibit higher scattering intensity for the anion when the outermost atomic columns of the tip are analyzed ( Fig. 3b , curve b2). The details of Z-contrast analysis are illustrated in Supplementary Fig. 3 . 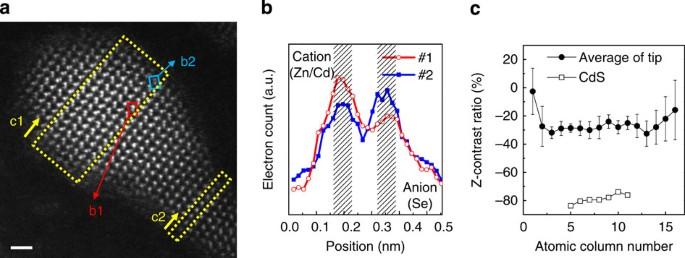Figure 3: High-resolution aberration-corrected STEM analysis of ZnSe shell (a) STEM image of a CdS/CdSe/ZnSe DHNR. Scale bar, 1 nm. (b) Z-contrast intensity of representative individual cation–anion column pairs—labelled b1 (CdSe-rich center of the tip) and b2 (mixed CdSe and ZnSe outer region of the tip) in (a). (c) Z-contrast intensity analysis of cation and anion column pairs along the perpendicular direction to the rod axis. Filled circles correspond to the average of all line scans of cation/anion pair columns along the direction of the arrow inside dotted rectangle labeled c1 in the STEM image of (a). Open squares correspond to the direction indicated for dotted rectangle labeled c2 in the STEM image of (a). Z-contrast is defined as (Ianion−Ication)/Ication, whereIjis the count of scattered electrons for ion column j. Figure 3c , curve c1 is the average of line scans of normalized cation–anion pair Z-contrast across the center region of the tip. There appears to be Z-contrast inversion near the edges as expected in the presence of ZnSe where the cation is now the lighter element. Line scans of cation–anion pairs across the CdS region of the DHNR shows no obvious sign of ZnSe growth ( Fig. 3c , curve c2). We note that each scattering peak corresponds to an entire column of atoms, and therefore we can expect a mixture of CdSe and ZnSe over the entire tip region. Furthermore, reduced signal-to-noise ratio at the edges, surface reconstruction and higher mobility of surface atoms may all complicate the observed signal. Therefore, despite the expectation of the outer edges of the tip having larger contributions from ZnSe, not all edge signals exhibit Z-contrast inversion and cause relatively large overlapping error bars in Fig. 3c . Nevertheless, these results combined with average diameter changes, EDS and XRD results provide a strong evidence for selective tip growth of a few monolayers of ZnSe. Figure 3: High-resolution aberration-corrected STEM analysis of ZnSe shell ( a ) STEM image of a CdS/CdSe/ZnSe DHNR. Scale bar, 1 nm. ( b ) Z-contrast intensity of representative individual cation–anion column pairs—labelled b1 (CdSe-rich center of the tip) and b2 (mixed CdSe and ZnSe outer region of the tip) in ( a ). ( c ) Z-contrast intensity analysis of cation and anion column pairs along the perpendicular direction to the rod axis. Filled circles correspond to the average of all line scans of cation/anion pair columns along the direction of the arrow inside dotted rectangle labeled c1 in the STEM image of ( a ). Open squares correspond to the direction indicated for dotted rectangle labeled c2 in the STEM image of ( a ). Z-contrast is defined as ( I anion − I cation )/ I cation , where I j is the count of scattered electrons for ion column j. Full size image Optical properties The absorption and PL spectral changes at each step of the synthesis provide interesting insights into both optical properties and composition/structure of the DHNRs. The bottom-most spectra in Fig. 4a correspond to the seed CdS nanorods. Both absorption and PL exhibit narrow linewidths indicative of a very narrow diameter distribution. In particular, band-edge emission peak near 470 nm has full width at half maximum (FWHM) of 16 nm (84 meV). The growth of the CdSe tips leads to a new absorption feature near 585 nm and the corresponding PL from CdSe band edge. The double-peaked PL spectrum of CdS/CdSe nanorod heterostructures arises from a bimodal size distribution of CdSe presumably owing to the differentiation of growth rates on the two ends of the seed CdS nanorod [30] , [40] , [41] (see Supplementary Fig. 4 ). The radial dimensions of the growing CdSe tips are within about a monolayer length of the seed CdS nanorod diameter, but the longitudinal dimension is what becomes bimodal. One of the tips has a length along the rod axis that is smaller than the rod diameter leading to the shoulder in the PL spectrum near 560 nm. PL excitation spectra measured at two different emission wavelengths corresponding to two different CdSe sizes exhibit same CdS contributions indicating that both are attached to CdS seed nanorods rather than isolated particles (see Supplementary Fig. 4 ). The two different growth rates may be exploited to develop single-tipped DHNRs. Interestingly, the bimodal size distribution of CdSe does not cause significant line broadening in the final DHNRs. After ZnSe growth, we have observed emission intensity to increase up to ~15 times while a narrow single-emission peak emerges. FWHM of DHNRs as narrow as 24 nm (80 meV) has been observed (for the case of shown in Fig. 4a second spectrum from top, FWHM is ~29 nm or 96 meV). As a comparison, the best CdSe/CdS core/shell QDs of similar emission wavelength show 20–30 nm PL FWHM [42] , [43] . The convergence of the two CdSe PL peaks may be a result of enhanced growth of ZnSe on the smaller CdSe tip, which in turn would lead to a larger redshift than the PL of the larger CdSe tip on ZnSe shell growth [44] . The 15-fold increase in PL while maintaining narrow linewidth and the narrow size distribution of the seed CdS nanorod despite the two-step growth is highly promising for developing more complex heterostructures. 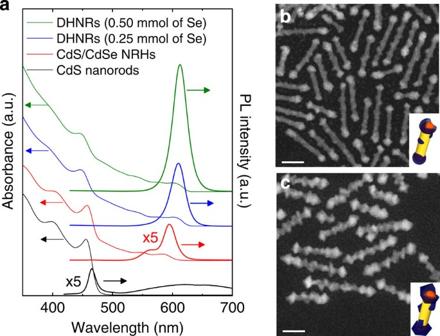Figure 4: The evolution of optical properties and geometric shape with ZnSe thickness. (a) From bottom to top, absorption and emission spectra of CdS nanorods, CdS/CdSe nanorod heterostructures and CdS/CdSe/ZnSe DHNRs of two different ZnSe amounts. (b,c) STEM images of different thickness of ZnSe grown on CdS/CdSe nanorod heterostructures. Scale bar, 20 nm. Figure 4: The evolution of optical properties and geometric shape with ZnSe thickness. ( a ) From bottom to top, absorption and emission spectra of CdS nanorods, CdS/CdSe nanorod heterostructures and CdS/CdSe/ZnSe DHNRs of two different ZnSe amounts. ( b , c ) STEM images of different thickness of ZnSe grown on CdS/CdSe nanorod heterostructures. Scale bar, 20 nm. Full size image Figure 4a shows that continued ZnSe growth by injecting additional Se precursor leads to a further improvement in PL (reaching up to 39% absolute PL quantum yield so far without any other optimization, for example, by choosing different surface-capping molecules). The increasing absolute PL yield with increasing Se precursor amount for ZnSe growth and therefore ZnSe thickness is shown in Supplementary Fig. 5 . In the core/shell nanocrystals, continued shell growth can lead to decreasing PL yields due to lattice strain buildup [19] . Figure 1f,g and 4b,c as well as additional STEM and EDS analyses (see Supplementary Fig. 6 ) indicate that ZnSe initially grows selectively on CdSe tips but eventually grows on the sides of the CdS seed nanorods. The continued increase in PL yields may then be explained by the passivation of CdS surface traps by ZnSe. Since the linewidth and the wavelength of the PL do not change, we conclude that the appearance of type II emission across the CdS/ZnSe interface is negligible. Furthermore, this side growth is not continuous and therefore maintains physical access to CdS, which will be beneficial for carrier injection and extraction processes. LEDs Having established the double-heterojunction structure that allows high PL quantum yields with narrow linewidths, we now discuss the impact of the staggered band offset of CdS and ZnSe by examining the electroluminescence (EL) performance of DHNRs. LEDs with DHNRs as emitting elements (DHNR LEDs) were fabricated with device design similar to reported core/shell nanocrystal LEDs (C/S LEDs) [9] , [45] , [46] . 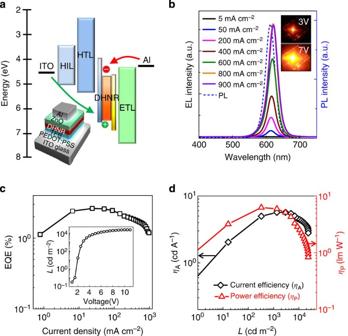Figure 5: Device structure and characteristics of the DHNR LEDs. (a) Energy band diagram of the DHNR LED along with a schematic of device structure. (b) EL spectra of a DHNR LED at the indicated applied current densities plotted along with the normalized PL spectrum of the DHNR film and photographs of a working device operating at the indicated voltages. (c) External quantum efficiency versus current density. Inset shows the dependence of luminance (L) on the applied voltage. (d) Dependence of current and power efficiencies onL. Figure 5a inset shows the schematic of our device structure. A cross-sectional TEM image is shown in Supplementary Fig. 7a . The device consists of a pre-patterned indium tin oxide (ITO) anode and poly(ethylenedioxythiophene):poly(styrenesulphonate) as the hole injection layer, poly[(9,9-dioctylfluorenyl-2,7-diyl)-co-(4,40-(N-(4-sec-butylphenyl)) diphenylamine)] (TFB) as the hole transport layer, DHNRs as the emissive layer, ZnO as the electron transport layer (ETL) and an electron-beam evaporated Al layer as the cathode. The DNHR emissive layer is ~25 nm thick, which is less than the average length of the nanorods. This thickness and the SEM images of the DHNR film (see Supplementary Fig. 7b ) suggest that DHNRs are primarily orientated parallel to the device plane. The transport layers and electrodes used here have also been used in C/S LEDs with external quantum efficiencies (EQEs) reaching up to ~1.7% for emission wavelength comparable to our DHNR LEDs [9] , [45] , [46] . Figure 5a shows the energy band diagram of our DHNR LEDs that should lead to efficient carrier injection to the DHNRs (especially for holes) owing to the presence of the double heterojunction. Figure 5b shows the PL spectrum of our DHNR in film (dashed line) and EL spectra of the corresponding DHNR LED at the indicated current densities. Slight redshift of EL spectra compared with the PL spectrum can be seen with increasing current densities, which is expected based on the well-known Stark effect [47] . The DHNR LEDs exhibit even narrower EL peak width (FWHM 29 nm, 96 meV) than previous C/S LEDs (38~39 nm, 115~131 meV) for EL peak position 600~640 nm [9] , [10] . Furthermore, no parasitic emission from the adjacent layers (that is, TFB or ZnO) is observed over the entire device operation range (see Fig. 5b ). Figure 5: Device structure and characteristics of the DHNR LEDs. ( a ) Energy band diagram of the DHNR LED along with a schematic of device structure. ( b ) EL spectra of a DHNR LED at the indicated applied current densities plotted along with the normalized PL spectrum of the DHNR film and photographs of a working device operating at the indicated voltages. ( c ) External quantum efficiency versus current density. Inset shows the dependence of luminance ( L ) on the applied voltage. ( d ) Dependence of current and power efficiencies on L . Full size image Compared with the previously reported C/S LEDs using a similar device architecture, our devices exhibit lower threshold voltage (~1.3 V if defined as the point of the steep rise at the beginning of trap-limited conduction regime or ~1.6 V if defined as the driving voltage corresponding to a luminance of 0.1 cd m −2 ) [8] , [9] , [45] , [48] . The maximum luminance of the DHNR LED shown in Fig. 5c inset is 31,010 cd m −2 . The highest brightness we have observed in DHNR LEDs is 36,000 cd m −2 . The maximum EQE of DHNR LEDs measured thus far is 2.62% ( Fig. 5c ), and the corresponding maximum current and power efficiencies are 5.70 cd A −1 and 6.26 lm W −1 , respectively ( Fig. 5d ). These values represent significant improvements over the best reported C/S LEDs using similar device architecture and emission wavelength [9] , [45] , [46] (cf. maximum values of brightness=31,000 cd m −2 , EQE=1.7%, current efficiency=3.9 cd A −1 and power efficiency=3.8 lm W −1 for orange/red emitting C/S LEDs in ref. 9 ) and nearly an order of magnitude brighter and a factor of 4 higher in maximum EQE than the only other ‘nonspherical’ nanocrystal-based LEDs recently reported [49] . As shown in Supplementary Fig. 5 , increasing ZnSe thickness leads to improved PL yields, which directly translates to EQE improvements. This observation is consistent with our earlier suggestion that, the partial side growth ZnSe on CdS still allows efficient electron injection into CdS while allowing the benefit of passivating CdS surface traps. Given that our devices simply ‘borrow’ carrier injection and transport layers established for core/shell nanocrystals without any significant materials or thickness optimization for the new emissive layer (for example, thickness and orientation of nanorod film, proper materials choice for the transport layers and so on) and that the PL of our yet-to-be optimized DHNRs reach only up to ~40%, whereas the core/shell nanocrystals typically reach PL yields of ~80%, these achieved performances are especially noteworthy. As impressive are the low turn-on voltage, narrow EL bandwidth and the stability under air ambient operation (see Supplementary Fig. 8 ), which represent additional improvements over the best C/S LEDs with a similar device architecture reported to date [9] , [10] . These promising characteristics of DHNR LEDs support our speculation that incorporation of double heterojunctions into the emitting nanocrystals can facilitate/enhance carrier injection processes. The DHNRs achieved here represent the beginning of a new subclass of nanocrystals that incorporate both type I and type II band offsets, where the heterojunctions are active rather than passive insulators. Specifically shown here is the case of two distinct materials both in contact with one CdSe QD-facilitating electron and hole injection (and blocking of opposite charge carriers) independently. This type of ability to engineer band structure/offsets via functional heterojunctions with spatial anisotropy in colloidal nanorods affords exciting prospects for utilizing solution-processable nanomaterials for high-performance devices. As an example, we have demonstrated LEDs incorporating our DHNRs as emissive layers. These devices exhibit narrow EL bandwidths, low threshold voltages and stability under air operation with efficiencies superior to the current state-of-the-art C/S LEDs using similar device architecture. Given the recent finding of charging of CQDs from ETL reducing device efficiencies (for example, via multi-carrier Auger recombination) [50] , DHNRs with independently variable electron and hole injection barriers are excellent candidate materials for compensating or minimizing such loss mechanisms. Indeed, the lowered hole barrier through the use of ZnSe in our DHNRs may already be helping to balance charge in LED operation, but further studies are needed to verify. Fine-tuning of DHNR morphology (for example, transition from double tip growth to single tip growth) along with DHNR-specific optimization of device architecture (for example, optimizing assembly beyond the current random orientation of nanorods afforded by simple spin-casting and utilizing inverted device structure as recently demonstrated in refs 10 , 11 for C/S LEDs) should lead to further improvements in device performance. We anticipate such efforts to lead to broader applicability of DHNRs (for example, in photodetectors and photovoltaics). In general, building on our simple strategy to extend anisotropic nanorod growth to introduce the double heterojunction (while maintaining narrow size distribution) should pave the path for developing application-specific design and synthesis of multi-component, multi-functional nanoheterostructures. Materials Technical grade trioctylphosphine oxide (90%), technical grade trioctylphosphine (TOP) (90%), technical grade oleic acid (90%), technical grade octadecene (90%), CdO (99.5%), Zn acetate (99.99%), S powder (99.998%) and Se powder (99.99%) were obtained from Sigma Aldrich. N -octadecyl phosphonic acid (ODPA) was obtained from PCI Synthesis. ACS grade chloroform and methanol were obtained from Fischer Scientific. All chemicals were used as received. Synthesis of CdS nanorods CdS nanorods were prepared in a manner similar to established methods [14] . The reactions were carried out in a standard Schlenk line under N 2 atmosphere. First, 2.0 g (5.2 mmol) of trioctylphosphine oxide, 0.67 g (2.0 mmol) of ODPA and 0.13 g (2.0 mmol) of CdO in a 50-ml three-neck round-bottom flask were degassed at 150 °C for 30 min under vacuum, and then heated to 350 °C with stirring. As the Cd–ODPA complex was formed at 350 °C, the brown solution in the flask became optically transparent and colourless typically after 1 h. The solution was then cooled and degassed at 150 °C for 10 min to remove by-products of complexation including O 2 and H 2 O. After degassing, the solution was reheated to 350 °C under N 2 atmosphere. S precursor containing 16 mg (0.5 mmol) of S dissolved in 1.5 ml of TOP was swiftly injected into the flask with a syringe. Consequently, the reaction mixture was quenched to 330 °C where the CdS growth was carried out. After 15 min, the CdS nanorods growth was terminated by cooling to 250 °C, where the CdSe growth on CdS nanorods was carried out. An aliquot of the CdS nanorods was taken and cleaned by precipitation with methanol and butanol for characterization. The CdS/CdSe heterostructures were formed by adding Se precursor slowly to the same reaction flask, maintained under N 2 atmosphere as described below. Synthesis of CdS/CdSe nanorod heterostructures The one-pot synthesis of rod-rod-rod shaped nanorod heterostructures were carried out in a similar manner to the established method [31] , [36] . Following the formation of CdS nanorods, Se precursors containing 20 mg (0.25 mmol) of Se dissolved in 1.0 ml of TOP was slowly injected at 250 °C at a rate of 4 ml h −1 via syringe pump (total injection time ~15 min). The reaction mixture was then allowed to stir for an additional 5 min at 250 °C before being rapidly cooled by an air jet. An aliquot of CdS/CdSe nanorod heterostructures was taken and cleaned by precipitation with methanol and butanol for analysis. The final reaction mixture was dissolved in chloroform, and centrifuged at 2,000 r.p.m. The precipitate was redissolved in chloroform for the next step. This solution of CdS/CdSe nanorod heterostructures had an optical density of 0.75 (in a cuvette with 1 cm optical path length) at the CdS band-edge absorption peak when diluted by a factor of 10. Synthesis of CdS/CdSe/ZnSe DHNRs CdS/CdSe/ZnSe DHNRs were synthesized by growing ZnSe onto CdS/CdSe nanorod heterostructures. For Zn precursor, 6 ml of octadecene, 2 ml of oleic acid and 0.18 g (1.0 mmol) of Zn acetate were degassed at 150 °C for 30 min. The mixture was heated to 250 °C under N 2 atmosphere, and consequently Zn oleate was formed after 1 h. 2 ml of previously prepared CdS/CdSe stock solution was injected into Zn oleate solution after cooling to 50 °C. Chloroform was allowed to evaporate for 30 min under vacuum at 70 °C. ZnSe growth was initiated by a slow injection of the Se precursor containing 39 mg (0.50 mmol) of Se dissolved in 2.0 ml of TOP to the reaction mixture at 250 °C. Thickness of ZnSe on CdS/CdSe nanorod heterostructures was controlled by the amount of Se injected. The ZnSe growth was terminated by removing the heating mantle after injecting the desired amount of Se precursor. Cleaning procedures were same as described for the CdS nanorods. Device fabrication DHNR LEDs were fabricated on ITO-coated glass substrates (sheet resistance of 15~25 Ω□ −1 ). The pre-patterned ITO substrates were cleaned with acetone and isopropanol, consecutively, and then treated with ultraviolet-ozone for 15 min. Poly(ethylenedioxythiophene):poly(styrenesulphonate) (Clevios P VP AI 4083), the hole injection layer was spin-coated onto the ITO at 4,000 r.p.m. and baked at 120 °C for 5 min in air and 180 °C for 15 min in an argon glove box. Then TFB (H.W. Sands Corp.) as a hole transport layer was spin-coated using m-xylene (0.5 mg ml −1 ) at 3,000 r.p.m., followed by baking at 180 °C for 30 min in an argon glove box. After washing twice with chloroform and methanol mixture (1:1 volume ratio), CdS/CdSe/ZnSe DHNRs were finally dispersed in chloroform solution (~30 mg ml −1 ), and spin-cast on top of the TFB layer at 500 r.p.m., and then subsequently annealed at 180 °C for 30 min in a glove box. ZnO as ETL (~30 mg ml −1 in butanol) was spin-coated at 3,000 r.p.m. and annealed at 100 °C for 30 min. ZnO nanoparticles were synthesized following the literature [51] . A solution of potassium hydroxide (1.48 g) in methanol (65 ml) was added to zinc acetate dihydrate (2.95 g) in methanol (125 ml) solution and the reaction mixture was stirred at 60 °C for 2 h. The mixture was then cooled to room temperature and the precipitate was washed twice with methanol. After ZnO spin-casting, an ~100-nm-thick Al cathode was deposited by an electron-beam evaporator at a rate of 1 Å s −1 . Finally, the devices were encapsulated using a cover glass with epoxy (NOA 86) in a glove box. Characterization TEM samples were prepared on Cu grids with thin carbon film from a dilute solution of nanorods in chloroform. TEM analysis was carried out with a JEOL 2100 TEM operating at 200 kV. EDS and STEM analyses were carried out with a JEOL 2200 aberration-corrected STEM/TEM operating at 200 kV. HAADF STEM images were obtained with ~100 mrad of HAADF inner cutoff angle, 26.61 mrad of beam convergence half angle and 30 pA of probe current. Ultraviolet–visible absorption spectra were obtained with an Agilent 8453 photodiode array spectrometer. PL spectra were collected with a Horiba Jobin Yvon FluoroMax-3 fluorometer. The absolute PL quantum yield was obtained using a Quantamaster 40 spectrophotometer. DHNRs dispersed in toluene were dispensed in a 4-ml rectangular quartz cuvette and inserted into a sample holder within a dark sample chamber. Emission spectrum was obtained using a fixed excitation wavelength (450 nm) and the emission wavelength was scanned between 400 and 800 nm with a 0.5-nm step size and integration time of 0.1 s. J–V and L–V characteristics, lifetime measurements and EL spectra were recorded using a Spectrascan PR-655 spectrophotometer coupled with a Keithely 2602B voltage and current source measurement unit. EQE can be calculated by the ratio of the number of photons emitted by the device to the number of electrons injected. Current and power efficiencies are defined as the ratio of the output luminance to the driving current density, and the ratio of the luminous flux output of the device to the corresponding driving electrical power, respectively. All device measurements including lifetime test were performed under air ambient conditions. How to cite this article: Oh, N. et al. Double-Heterojunction Nanorods. Nat. Commun. 5:3642 doi: 10.1038/ncomms4642 (2014).